The origin of the bifurcated axial skeletal system in the twin-tail goldfish Twin-tail goldfish possess a bifurcated caudal axial skeleton. The scarcity of this trait in nature suggests that a rare mutation, which drastically altered the mechanisms underlying axial skeleton formation, may have occurred during goldfish domestication. However, little is known about the molecular development of twin-tail goldfish. Here we show that the bifurcated caudal skeleton arises from a mutation in the chordin gene, which affects embryonic dorsal–ventral (DV) patterning. We demonstrate that formation of the bifurcated caudal axial skeleton requires a stop-codon mutation in one of two recently duplicated chordin genes; this mutation may have occurred within approximately 600 years of domestication. We also report that the ventral tissues of the twin-tail strain are enlarged, and form the embryonic bifurcated fin fold. However, unlike previously described chordin -deficient embryos, this is not accompanied by a reduction in anterior–dorsal neural tissues. These results provide insight into large-scale evolution arising from artificial selection. The vertebrate tail is supported by the caudal axial skeleton [1] , [2] . The axial skeletal system comprises several midline-located vertebral elements, and this basic architecture is highly conserved among vertebrates [1] , [2] . In addition, although teleost caudal fins exhibit divergent and complex skeletal elements, their basic architecture is fundamentally the same, with the fin ray and vertebral elements being located on the sagittal plane [1] , [2] , [3] , [4] ( Fig. 1a–d ). However, this highly conserved architecture has undergone drastic modification in certain goldfish ( Carassius auratus ) lineages, through artificial selection [5] , [6] , [7] , [8] , [9] , [10] ( Fig. 1e–j ). Several goldfish strains have been established for ornamental purposes [5] , [6] , [10] . Some of these strains, known as twin-tail goldfish, possess bifurcated caudal fins in which several caudal vertebral elements and their attaching fin-rays are duplicated to form a laterally bifurcated caudal axial skeletal system [7] , [8] , [9] ( Fig. 1e–i ). 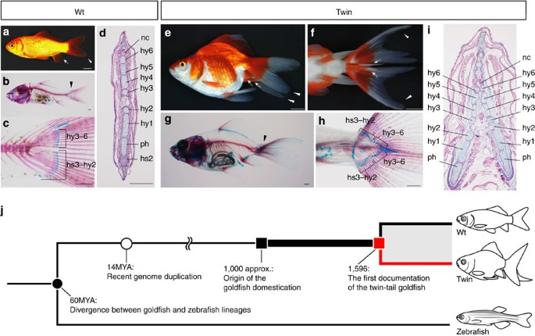Figure 1: Evolution of goldfish morphology. (a) Lateral view of the wild-type goldfish (Wt). (b) Skeletal structure of Wt goldfish. (c) Magnified view of the caudal region of the specimen inb. (d) Transverse section of the Wt at the caudal level. (e) Lateral view of the twin-tail goldfish (Twin). (f) Ventral view of the caudal region of the specimen ine. (g) Skeletal structure of Twin goldfish. (h) Magnified view of the ventral side of the specimen ing. (i) Transverse section of the Twin goldfish specimen. The approximate levels of sectioning are indicated by black arrowheads (b,g). Anal and caudal fins are indicated by white arrows and arrowheads, respectively (a,e,f). (j) Evolutionary events in the goldfish lineage. The black circle indicates the time of divergence between the goldfish and zebrafish lineages, and the white circle indicates the estimated time of the genome duplication in goldfish18. The red line represents the twin-tail goldfish lineage. hs, haemal spines; hy, hypural; MYA, million years ago; nc, notochord; ph, parhypural. Scale bars, 1 cm (a,e,f), 1 mm (b,c,g,h), 100 μm (d,i). Figure 1: Evolution of goldfish morphology. ( a ) Lateral view of the wild-type goldfish (Wt). ( b ) Skeletal structure of Wt goldfish. ( c ) Magnified view of the caudal region of the specimen in b . ( d ) Transverse section of the Wt at the caudal level. ( e ) Lateral view of the twin-tail goldfish (Twin). ( f ) Ventral view of the caudal region of the specimen in e . ( g ) Skeletal structure of Twin goldfish. ( h ) Magnified view of the ventral side of the specimen in g . ( i ) Transverse section of the Twin goldfish specimen. The approximate levels of sectioning are indicated by black arrowheads ( b , g ). Anal and caudal fins are indicated by white arrows and arrowheads, respectively ( a , e , f ). ( j ) Evolutionary events in the goldfish lineage. The black circle indicates the time of divergence between the goldfish and zebrafish lineages, and the white circle indicates the estimated time of the genome duplication in goldfish [18] . The red line represents the twin-tail goldfish lineage. hs, haemal spines; hy, hypural; MYA, million years ago; nc, notochord; ph, parhypural. Scale bars, 1 cm ( a , e , f ), 1 mm ( b , c , g , h ), 100 μm ( d , i ). Full size image Documented accounts of twin-tail goldfish first appear in Ming dynasty archives in 1,596 common era; furthermore, analysis of Chinese archives indicate that goldfish domestication began at around 1,000 common era in Song dynasty China [5] , [6] . Such historical accounts suggest that twin-tail goldfish emerged after approximately 600 years of domestication (bold line in Fig. 1j ), and the laterally bifurcated axial skeletal system has been subsequently maintained (red line in Fig. 1j ). The paucity of laterally bifurcated caudal axial skeletons in nature suggests that a rare mutation may have occurred during 600 years of goldfish domestication [8] , [11] , which drastically modified the developmental mechanisms underlying axial skeletal formation. In this study we identify the genetic alterations that gave rise to twin-tail goldfish, by conducting backcross analysis, functional assays and analysis of gene expression patterns. The results suggest that the bifurcated caudal fin morphology of twin-tail goldfish is caused by ventralization of early embryonic development, which is in turn due to a mutation in a chordin gene that may have arisen during the aforementioned domestication period [5] , [6] . Comparison between twin-tail goldfish and the dino zebrafish The phylogenetic and embryological similarity of goldfish and zebrafish suggest the possible existence of a zebrafish mutant with a phenotype similar to that of twin-tail goldfish [12] , [13] , [14] , [15] , [16] ( Fig. 1j ). To identify such a mutant, we compared embryonic and adult twin-tail goldfish with previously identified zebrafish fin mutants [7] , [8] , [9] , [14] , [16] . We report that twin-tail goldfish share three characteristic phenotypes (accumulation of blood cells, bifurcated fin folds and skeletal defects in the vertebral column) with the dino zebrafish mutant; the mutated gene in the dino mutant is chordin , a key player in DV patterning [7] , [14] , [17] , [18] , [19] , [20] , [21] , [22] ( Fig. 2a and Supplementary Figs 1 and 2 ). 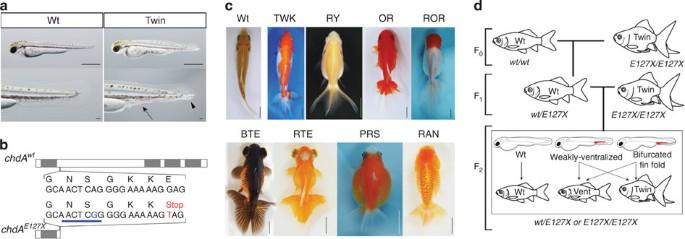Figure 2: The involvement of thechdAgene in the twin-tail phenotype. (a) Lateral view of wild-type (Wt) and twin-tail (Twin) goldfish larvae. The lower panels are magnified views of the larval caudal regions. Blood cell accumulation and duplicated fin folds are indicated by the black arrow and arrowhead, respectively. (b) The goldfishchdAwtand chdAE127Xamino-acid sequences. The positions of CR domains are indicated by grey boxes. The twin-tail-specific mutation changes a glutamic acid codon (GAG) to a stop codon (TAG) at amino-acid position 127 (the mutated nucleotide is indicated by the red ‘T’). A twin-tail-specificAvaI site is located near the stop codon (indicated by the blue line and ‘G’). (c) Dorsal views of the Wt and eight twin-tail goldfish strains. (d) Schematic detailing the phenotyping of backcross segregants. Scale bars, 1 mm (upper row ina), 0.1 mm (bottom row ina), approximately 1 cm (c). Figure 2: The involvement of the chdA gene in the twin-tail phenotype. ( a ) Lateral view of wild-type (Wt) and twin-tail (Twin) goldfish larvae. The lower panels are magnified views of the larval caudal regions. Blood cell accumulation and duplicated fin folds are indicated by the black arrow and arrowhead, respectively. ( b ) The goldfish chdA wt and chdA E127X amino-acid sequences. The positions of CR domains are indicated by grey boxes. The twin-tail-specific mutation changes a glutamic acid codon (GAG) to a stop codon (TAG) at amino-acid position 127 (the mutated nucleotide is indicated by the red ‘T’). A twin-tail-specific Ava I site is located near the stop codon (indicated by the blue line and ‘G’). ( c ) Dorsal views of the Wt and eight twin-tail goldfish strains. ( d ) Schematic detailing the phenotyping of backcross segregants. Scale bars, 1 mm (upper row in a ), 0.1 mm (bottom row in a ), approximately 1 cm ( c ). Full size image To examine whether the chordin gene is involved in the twin-tail goldfish phenotype, we isolated and sequenced its homologues from goldfish embryonic cDNA. We report that goldfish has at least two closely related chordin genes (designated as chdA and chdB ), which may be a consequence of a recent genome duplication [12] ( Fig. 1j and Supplementary Fig. 3 ). As for other vertebrate chordin genes, these two goldfish chordin paralogues encode four conserved cysteine-rich (CR) domains, which are important for the BMP antagonist and dorsal organizer roles of the proteins [18] , [21] , [22] , [23] . More significantly, we identified two alleles of the chdA gene; one allele (designated as chdA wt ) contains the wild-type codon at the 127th amino-acid site, while the second allele (designated as chdA E127X ) contains a stop codon at the same position ( Fig. 2b and Supplementary Fig. 3 ). The stop codon in chdA E127X is predicted to result in a truncated protein lacking the second to fourth CR domains ( Fig. 2b , Supplementary Fig. 3 ). Sequencing of PCR amplicons revealed that eight different twin-tail goldfish strains are homozygous for chdA E127X , while all allelic combinations were observed in wild-type goldfish populations ( Fig. 2c and Supplementary Fig. 4 ). These results suggest that the chdA E127X allele may contribute to the twin-tail phenotype in goldfish. Backcross analysis To investigate whether chdA E127X genetically correlates with the twin-tail phenotype, we analysed their association in backcross progeny ( Fig. 2d and Supplementary Fig. 5 ). The larval and juvenile stage phenotypes of a total of 670 backcross progeny were divided into the following three categories: wild-type ( n =333), vent ( n =41), and twin-tail ( n =296) ( Fig. 2d , Supplementary Figs 1 and 5 , Table 1 ). Progeny exhibiting the various phenotypes were genotyped using an allele-specific restriction site polymorphism ( Fig. 2b and Table 1 ). All 296 twin-tail specimens were homozygous for the chdA E127X specific site ( Fig. 2d and Table 1 ). Although the influence of other genes and environmental factors remains to be addressed, our genotyping results strongly suggest that homozygosity for the chdA E127X allele is essential for the development of the bifurcated axial skeletal system in twin-tail goldfish ( Fig. 2c,d and Table 1 ). Table 1 Phenotypes and genotypes of backcross progeny. Full size table Functional analysis of chdA To confirm the causal relationship between the chdA E127X allele and the twin-tail phenotype, we conducted rescue experiments using chdA wt mRNA ( Fig. 3 and Supplementary Fig. 6 ). Injection of chdA wt mRNA into twin-tail goldfish embryos resulted in a dose-dependent rescue of the phenotype ( Fig. 3a–e and Supplementary Fig. 6 ). Injection with 125 pg chdA wt mRNA rescued over 40% of embryos in a reproducible manner; three independent experiments using different clutches of embryos produced similar results ( n =176) ( Fig. 3e and Supplementary Fig. 6 ). The caudal skeletal morphology of the rescued goldfish individuals was almost identical to that of the wild type at the juvenile stage ( Figs 1a–c and 3f–j ). In contrast to chdA wt , injection of chdA E127X mRNA did not affect the twin-tail phenotype in any specimens ( Fig. 3e ). These results suggest that the chdA E127X allele causes the twin-tail goldfish phenotype. 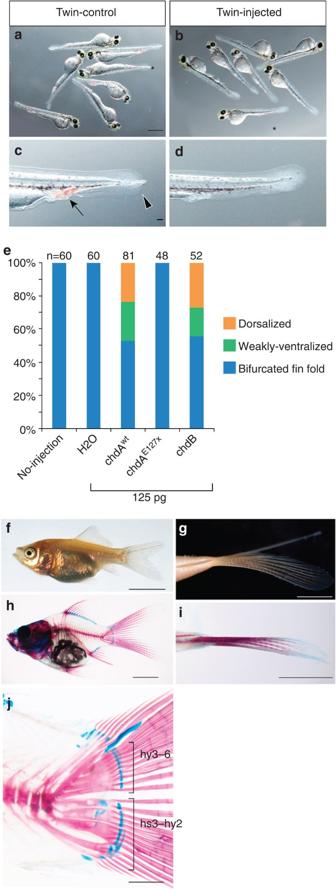Figure 3: Rescue of the twin-tail phenotype by mRNA microinjection. (a,b) Larval phenotypes of twin-tail goldfish. Non-injected controls (a) or embryos injected with 125 pgchdAwtmRNA (b). (c,d) Magnified view of the caudal regions indicated by asterisks inaandb, respectively. Arrow and arrowhead indicate accumulated blood cells and bifurcated fin folds, respectively. (e) Proportion of rescued specimens following injection of embryos with the indicated mRNA. The number of larvae analysed is indicated above each bar. (f–j) Twin-tail goldfish juvenile injected withchdAwtmRNA. (f) Lateral view. (g) Ventral view of the caudal level. (h) Lateral view of the skeletal structure. (j) Magnified view of the caudal region ofh. The dorsal phenotype criteria were based on previous descriptions. Panelsaandb, andcanddare at the same magnification, respectively. Scale bars, 1 mm (a,h,j), 100 μm (c), 5 mm (f–i). Figure 3: Rescue of the twin-tail phenotype by mRNA microinjection. ( a , b ) Larval phenotypes of twin-tail goldfish. Non-injected controls ( a ) or embryos injected with 125 pg chdA wt mRNA ( b ). ( c , d ) Magnified view of the caudal regions indicated by asterisks in a and b , respectively. Arrow and arrowhead indicate accumulated blood cells and bifurcated fin folds, respectively. ( e ) Proportion of rescued specimens following injection of embryos with the indicated mRNA. The number of larvae analysed is indicated above each bar. ( f – j ) Twin-tail goldfish juvenile injected with chdA wt mRNA. ( f ) Lateral view. ( g ) Ventral view of the caudal level. ( h ) Lateral view of the skeletal structure. ( j ) Magnified view of the caudal region of h . The dorsal phenotype criteria were based on previous descriptions. Panels a and b , and c and d are at the same magnification, respectively. Scale bars, 1 mm ( a , h , j ), 100 μm ( c ), 5 mm ( f – i ). Full size image Partial redundancy of chdA and chdB expression The similarity between the chdA and chdB sequences ( Supplementary Fig. 3 ) suggests they may have redundant functions, potentially implicating chdB in the twin-tail goldfish phenotype as well. To examine this hypothesis, we compared the function and expression patterns of the chdA and chdB genes in goldfish embryos ( Figs 3e and 4a,b , and Supplementary Fig. 7 ). We observed that injection of twin-tail goldfish embryos with either chdA wt or chdB mRNA resulted in similar levels of rescue, suggesting that these two chordin genes have a similar function ( Fig. 3e ). In addition, the chdA and chdB genes showed overlapping expression patterns in the dorsal-animal side of wild-type embryos during the middle gastrula stage (20–30% blastopore closure (bc) stages) ( Fig. 4a,b and Supplementary Fig. 7 ). Moreover, the expression patterns of chdB in wild-type and twin-tail goldfish embryos are similar ( Supplementary Fig. 7 ), suggesting that chdB plays a role in DV patterning in twin-tail embryos. Most significantly, the chdA gene exhibited a broader expression pattern than the chdB gene at the dorsolateral side of the blastoderm margin in gastrula embryos ( Fig. 4a,b ). These partially overlapping expression patterns suggest the chdB gene may compensate in part for the absence of chdA wt in twin-tail goldfish. 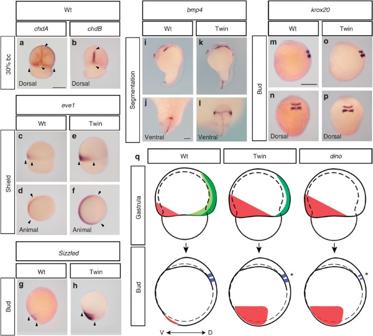Figure 4: Comparison of gene expression patterns between wild-type and twin-tail goldfish. (a–p) Expression patterns ofchdA(a),chdB(b),eve1(c–f),sizzled(g,h),bmp4(i–l) andkrox20(m–p). Unless otherwise noted, panels show lateral views of embryos. Black arrowheads indicate areas of gene expression. (j,l) Magnified views ofiandk, respectively. (q) Schematic representation of the gene expression patterns in wild-type and twin-tail goldfish, anddinozebrafish mutants. Light green, dark green, red and blue regions represent areas positive forchdAwt,chdB, ventral markers (eve1,sizzledandbmp4) andkrox20, respectively. Asterisks indicatekrox20expression areas in twin-tail goldfish anddinozebrafish. Panelsa–k,jandl, andm–pare at the same magnification. Scale bars, 500 μm (a,m); 100 μm (j). Figure 4: Comparison of gene expression patterns between wild-type and twin-tail goldfish. ( a – p ) Expression patterns of chdA ( a ), chdB ( b ), eve1 ( c – f ), sizzled ( g , h ), bmp4 ( i – l ) and krox20 ( m – p ). Unless otherwise noted, panels show lateral views of embryos. Black arrowheads indicate areas of gene expression. ( j , l ) Magnified views of i and k , respectively. ( q ) Schematic representation of the gene expression patterns in wild-type and twin-tail goldfish, and dino zebrafish mutants. Light green, dark green, red and blue regions represent areas positive for chdA wt , chdB , ventral markers ( eve1 , sizzled and bmp4 ) and krox20 , respectively. Asterisks indicate krox20 expression areas in twin-tail goldfish and dino zebrafish. Panels a – k , j and l , and m – p are at the same magnification. Scale bars, 500 μm ( a , m ); 100 μm ( j ). Full size image DV patterning of twin-tail goldfish embryos To more precisely determine how the functional redundancy and partially overlapping expression patterns of the goldfish chordin genes contribute to DV patterning in twin-tail embryos, we examined the expression patterns of ventral embryonic tissue markers ( eve1 , sizzled and bmp4 ) and a hindbrain marker gene ( krox20 ) ( Fig. 4c–p ) [19] , [20] , [24] , [25] . During the early-to-middle gastrula stage (shield to 30% bc stages), eve1 , sizzled and bmp4 showed overt ventralized expression patterns in twin-tail embryos ( Fig. 4c–f and Supplementary Fig. 7 ). Similarly, during the late gastrula (40% bc) to bud stages, these genes showed wider expression patterns in twin-tail than in wild-type embryos at posterior–ventral regions ( Fig. 4g,h and Supplementary Fig. 7 ). Moreover, bifurcated expression patterns of bmp4 were observed in the posterior region of twin-tail embryos during the segmentation stages ( Fig. 4i–l and Supplementary Fig. 7 ). These ventral marker expression patterns resemble those of dino zebrafish mutants and other chordin -deficient embryos [17] , [18] , [19] , [20] , [24] , [26] , [27] . In contrast to expression of these ventral markers, krox20 expression was no different between wild-type and twin-tail embryos at the bud stage ( Fig. 4m–p ), despite reports of it being significantly reduced in chordin -deficient vertebrate embryos [18] , [24] , [26] , [27] , [28] . Collectively, these results suggest that the absence of chdA wt during the gastrula stage causes an increase in ventral tissues in the posterior embryonic region ( Fig. 4c–h ), which in turn bilaterally shifts the fin fold primordial region ( Fig. 4i–l ); however, the presence of chdB prevents a reduction in dorsal–anterior tissues, such as the hindbrain ( Fig. 4m–p ). In summary, the partially overlapping expression patterns of chdA and chdB appear to enable wild type-like anterior–dorsal tissues and dino -like ventralized gene expression patterns to coexist in twin-tail embryos ( Figs 1j and 4q ). The finding that several morphologically and genetically divergent twin-tail goldfish strains are homozygous for the chdA E127X allele suggests that this genotype was selected during 600 years of domestication [6] , [10] , [29] (bold line, Figs 1j and 2b,c and Supplementary Fig. 4 ), and became fixed in the common ancestor of twin-tail strains [5] , [6] (red box, Fig. 1j ). The low reported survival rate for chordin teleost mutants suggests that homozygous chordin mutants may not readily emerge in a natural (or even artificial) environment [20] , [27] . In fact, it was reported that only 13% of dino zebrafish survived up to 7 days post fertilization (dpf) [20] . However, our backcross segregation experiments revealed that non-wild-type goldfish embryos (weakly-ventralized and bifurcated fin fold) are no less viable than their wild-type counterparts; over 70% of both mutant and wild-type embryos survived up to 9 dpf ( Fig. 2d and Supplementary Table 1 ). Although it is still unknown whether the common ancestor of twin-tail goldfish also exhibited such a high survival rate, these results lead us to hypothesize that the duplication of the chordin gene, and the overlapping expression patterns of the resulting paralogues ( Fig. 4q ), may have enabled the emergence of twin-tail goldfish; these strains were subsequently established and maintained by breeders in Song to Ming dynasty, China, a time period lacking sophisticated aquarium systems [5] , [6] . The above results also provide insight into the evolution of the robust and highly conserved developmental mechanism controlling DV patterning [18] , [30] . Large-scale morphological changes, which require extensive modification of such developmental mechanisms, are often presumed to require a relatively long period of evolutionary time [1] , [2] . However, here we have identified that a dramatic morphological and developmental change occurred in goldfish in a period of only 600 years, as a consequence of a recent gene duplication and subsequent artificial selection ( Fig. 1j ). During artificial selection, it is possible that mutations other than chdA E127X may have accumulated, and some of these may contribute to the twin-tail goldfish phenotype [5] , [6] ( Fig. 1j ). In fact, our genotyping analyses revealed that the wild-type populations and wild-type individuals among the backcross segregants contain the chdA E127X/E127X locus, therefore indicating incomplete penetrance ( Supplementary Fig. 4 and Table 1 ). More significantly, we observed that some embryos demonstrating a weakly-ventralized and bifurcated fin fold phenotype ultimately developed into ‘wild type-like’ juveniles, designated as ‘Vent’ ( Fig. 2d , Table 1 , and Supplementary Fig. 5 ). These results suggest that additional genetic and/or environmental factors may suppress or enhance the effect of the chdA E127X allele during development. Although any such factors are yet to be identified, certain DV patterning-related genes are putative candidates [18] , [21] , [22] . We hope to identify the additional factors which have modified the robust molecular developmental mechanisms for DV patterning and axial skeletal morphology. Goldfish strains and maintenance Wild-type and twin-tail strain goldfish (duplicated caudal fin Wakin, Ryukin, Oranda, Redcap Oranda, Black telescope, Red telescope, Perl scale and Ranchu) were purchased from an aquarium fish agency and breeder in Taiwan. To avoid confusion derived from differences between the goldfish nomenclature systems used by breeders and researchers [6] , [10] , [31] , this study defined goldfish individuals with a slender body and a single fin as wild type. The nomenclature of the twin-tail goldfish strains primarily followed that of Smartt [6] . Anatomical and histological analyses of axial skeletons Cleaned skeletal samples were prepared by fixing juvenile goldfish specimens in 10% formalin. The specimens were subsequently washed in 70% ethanol, stained first with alcian blue staining solution (0.1% alcian blue in 99.8% ethanol:acetic acid=4:1) and then with alizarin red solution (0.1% alizarin red in 95% ethanol), and finally cleared using ScaleA2 (ref. 32 ). For histological analysis, Bouin-fixed juvenile goldfish specimens were embedded in paraffin, sectioned to 5 μm using a slicer (RM2245, Leica), and stained with Alcian blue, hematoxylin and eosin. The cleaned skeletal and histological samples were examined using stereo and standard microscopes (SZX16 and BX43, Olympus). Caudal axial skeletal elements were identified and described on the basis of earlier reports [1] , [2] , [3] , [4] , [7] , [9] . The research followed internationally recognized guidelines. We received ethical approval from Institutional Animal Care & Utilization Committee, Academia Sinica. Goldfish embryos Sperm was extracted from multiple male goldfish and preserved in Modified Kurokura’s extender 2 solution at 4 °C [33] . Eggs were squeezed from mature female goldfish onto Teflon-coated dishes. Artificial fertilization was performed using dry methods. Fertilized eggs were placed in 9 cm Petri dishes or 3 l aquarium tanks containing tap water (22–24 °C). Serial ID numbers were provided for male and female individuals used for artificial fertilization. Petri dishes containing approximately 50–100 individuals were incubated at 24 °C until observation and harvesting. Embryonic stages were determined using the goldfish staging table before harvesting [13] . Gastrula, segmentation, pharyngular and hatching stages were determined on the basis of blastopore closure, somite number, otic vesicle closure and pectoral fin shape, respectively [13] . Molecular cloning and sequencing Homologues of chdA , chdB , eve1 , sizzled , bmp4 and krox20 were isolated from wild-type goldfish embryo cDNA using PCR. Total RNA was extracted from wild-type gastrula stage embryos using TRIzol Reagent (Ambion). Degenerate and specific PCR primers were designed on the basis of conserved amino-acid sequences and RNA-seq data. Multiple amino-acid alignments were used to identify conserved regions. Total RNA was also subjected to RNA-seq analysis by the Beijing Genomics Institute (BGI, Shenzhen, China). The insert size of the sequencing library for RNA-seq was 200-bp, and the 90-bp pair-end raw reads were generated using an Illumina HiSeq2000. The zebrafish chordin , eve1 , sizzled , bmp4 and krox20 sequences were used as queries to BLAST search (blastn and tblastn) against the RNA-seq data for primer design. Primers used to clone goldfish genes are listed in Supplementary Table 2 . PCR fragments amplified using these primers were isolated and purified, and then ligated into vectors using the TOPO TA Cloning Kit Dual Promoter (Invitrogen), T&A Cloning Vector Kit (Yeastern Biotech) or pGEM-T Easy Vector system (Promega). The resulting vectors were used to transform Escherichia coli DH5α. Over 10 clones were picked from each population for sequencing. The sequenced cDNA fragments were used as backbones to obtain the almost-complete sequences by PCR, with specific primers and the GeneRacer kit (Invitrogen), according to the manufacturer’s protocol ( Supplementary Table 2 ). The isolated genes were identified by generating multiple amino-acid alignments of goldfish and orthologous genes using CLUSTALW [34] . The phylogenetic relationships of goldfish chordin genes were investigated by reconstructing maximum likelihood trees using MEGA5 (ref. 35 ). To identify candidate loci in the chdA and chdB genes responsible for the twin-tail goldfish phenotype, the complete coding regions were isolated and sequenced from wild-type and twin-tail goldfish embryonic cDNA ( Supplementary Table 2 ). Single-nucleotide polymorphisms were examined by visual inspection; this revealed a substitution at the first nucleotide of the codon encoding the 127th amino acid of chdA in twin-tail goldfish, which causes the stop codon mutation (designated as chdA E127X ). DNA fragments containing the mutation site were amplified from the genomic DNA of wild-type and twin-tail goldfish individuals by PCR, using a specific pair of primers (chda-f5 and chd-r5 in Supplementary Table 2 ). These PCR amplicons were sequenced directly using an ABI 3730. The goldfish RNA-seq data and chdA , chdB , eve1, sizzled, bmp4 and krox20 sequences have been deposited in NCBI under accession numbers DRA001224 , and AB874473 to AB874479 , respectively. Backcross lines In 2012, wild-type male goldfish ( chdA wt/wt ) were independently mated with two twin-tail goldfish females (Oranda and Ryukin strains; chdA E127X/E127X ) ( Supplementary Fig. 5 ). Two F 1 hybrid strains derived from the two crosses were maintained in aquaria (200–1,000 l) at the Yilan Marine Station, ICOB, Academia Sinica, and the Aquaculture Breeding Institute, Hualien, Taiwan. In 2013, two F 1 hybrid individuals (WO, the wild type × Oranda strain, and WR, the wild type × Ryukin strain; chdA wt/E127X ) were mated with twin-tail goldfish individuals ( chdA E127X/E127X ) to obtain two backcross strains (OR × WO and RY × WR). The pedigree diagram is shown in Supplementary Fig. 5 . Phenotyping of backcross segregants The backcross segregants were phenotyped at both the late embryonic and larval stages. In addition, mutant segregants and wild-type individuals were maintained separately, to prevent the loss of segregants to competition. Initially, embryos at 2–3 dpf were pre-categorized based on morphology at the post-cloacal levels ( Supplementary Figs 1 and 5 ) into three types: wild-type; weakly-ventralized; and bifurcated fin fold. At 9–10 dpf, these pre-categorized segregants were further categorized into three types: wild-type (Wt) larvae from wild-type embryos; single caudal fin (Vent) larvae from weakly-ventralized or bifurcated caudal fin fold embryos; and bifurcated caudal fin (Twin) larvae from weakly ventralized or bifurcated fin fold embryos ( Supplementary Fig. 5 ). The embryonic phenotypes were defined on the basis of earlier descriptions of zebrafish dino mutants [17] , [19] , and the larval phenotypes on the basis of the presence or absence of duplicated caudal skeletons. All backcross embryos and larvae were observed under stereomicroscopy (SZX16 and SZ16; Olympus). In total, 942 segregants were phenotyped at the embryonic stage and 670 of these segregants were phenotyped at larval stages. Genotyping of chdA in backcross segregants A total of 670 phenotyped specimens were genotyped by restriction digestion of genomic PCR products. PCR primers were designed to amplify the region containing both the twin-tail chdA E127X allele and the closely linked Ava I restriction enzyme site ( Fig. 2b and chda-f5 and chd-r5 in Supplementary Table 2 ). PCR fragments amplified by these specific primers were digested by Ava I, and separated on 2% agarose gels. Genotypes were determined on the basis of the resulting band patterns. Injection of mRNA To generate constructs for transcription, the coding regions of chdA wt , chdA E127X or chdB were amplified by PCR and cloned into the pCS2+ vector [36] . These constructs were digested with Not I, and used as templates to synthesize capped mRNA with the mMESSAGE mMACHINE SP6 Kit, according to the manufacturer’s instructions (Ambion Inc.). The synthesized mRNA transcripts were purified using Quick Spin Columns for purification of radiolabelled RNA (Roche), and resuspended in nuclease-free water. A microinjector (Eppendorf Femtojet; Eppendorf) was used to inject mRNA into the centre of the yolk of 1–2 cell stage fertilized eggs, maintained on Petri dishes in 2 nl of 0.2 M KCl. Phenol red (Sigma) was added as an indicator at a final concentration of 0.05%. The injected embryos were incubated at 24 °C. Three independent rescue experiments were performed by injecting chdA wt into twin-tail goldfish embryos ( Supplementary Fig. 6 ). Control embryo phenotypes were examined for all three experiments. All control embryos derived from two of three clutches possessed bifurcated fin folds ( Supplementary Fig. 6 ). At 2 days after injection, embryos were classified by morphological inspection into the following three categories: weakly-ventralized, bifurcated fin fold and dorsalized. Categorization of the weakly-ventralized and bifurcated fin fold was based on the post-cloacal morphology ( Supplementary Fig. 1 ). Embryos lacking part (or all of) the caudal fins were defined as dorsalized, with reference to descriptions of zebrafish mutant phenotypes [19] , [37] . In situ hybridization Digoxigenin-labelled anti-sense RNA probes were produced using PCR product as template, and the SP6/T7 RNA polymerase Riboprobe Combination System (Promega), in accordance with the manufacturer’s instructions. The probes were subsequently purified using mini Quick Spin RNA Columns (Roche). Primer sets used for the amplification of the PCR fragments are listed in Supplementary Table 2 . For eve1 , sizzled , bmp4 and krox20 , the PCR product used to generate the probe corresponds to the full-length coding region. To avoid non-specific hybridization resulting from the high similarity of the chdA and chdB transcripts, anti-sense probes against these chordin genes were synthesized from the sequences encompassing the 3′ untranslated regions. Whole-mount in situ hybridization was performed as previously described [38] , with minor modifications. Goldfish embryos were fixed with 4% paraformaldehyde in PBS overnight. Gastrula stage embryos were fixed and then dechorionated using forceps. Segmentation and pharyngeal stage embryos were dechorionated before fixation through pronase treatment. After fixation and dechorionation, embryos were dehydrated with methanol. Dehydrated embryos were re-hydrated with PBT and re-fixed with 4% paraformaldehyde in PBS. Embryos were subsequently treated with Proteinase K for 20 min, and then re-fixed again. Pre-hybridization and hybridization were performed at 65 °C for a period between 1 h and overnight. The samples were washed sequentially with 66% formamide/2 × SSCT at 65 °C for 30 min, 33% formamide/2 × SSCT at 65 °C for 30 min, 2 × SSCT at 65 °C for 15 min, and 0.2 SSCT at 65 °C for 30 min (this last wash was repeated twice). The samples were then incubated in blocking solution (PBS, 10% heat-inactivated goat serum (Roche), 0.1% Tween-20) for 1 h, before being incubated with a 1/4,000–1/8,000 volume of anti-digoxigenin-AP Fab fragments (Roche) at room temperature for 4 h or at 4 °C overnight. Samples were washed four times with blocking solution at room temperature for 25 min each. Signals were detected using BCIP/NBT Color Development Substrate (Promega). The reaction was stopped by washing the samples with PBS. To ensure accurate comparison of gene expression levels, the wild-type and twin-tail goldfish embryos were treated under identical conditions. Accession codes: The goldfish RNA-seq data and chdA , chdB , eve1, sizzled, bmp4 and krox20 sequences have been deposited in DDBJ/EMBL/GenBank under accession numbers DRA001224 , and AB874473 to AB874479 , respectively. How to cite this article: Abe, G. et al. The origin of the bifurcated axial skeletal system in the twin-tail goldfish. Nat. Commun. 5:3360 doi: 10.1038/ncomms4360 (2014).